Stomatal responses of terrestrial plants to global change Quantifying the stomatal responses of plants to global change factors is crucial for modeling terrestrial carbon and water cycles. Here we synthesize worldwide experimental data to show that stomatal conductance ( g s ) decreases with elevated carbon dioxide (CO 2 ), warming, decreased precipitation, and tropospheric ozone pollution, but increases with increased precipitation and nitrogen (N) deposition. These responses vary with treatment magnitude, plant attributes (ambient g s , vegetation biomes, and plant functional types), and climate. All two-factor combinations (except warming + N deposition) significantly reduce g s , and their individual effects are commonly additive but tend to be antagonistic as the effect sizes increased. We further show that rising CO 2 and warming would dominate the future change of plant g s across biomes. The results of our meta-analysis provide a foundation for understanding and predicting plant g s across biomes and guiding manipulative experiment designs in a real world where global change factors do not occur in isolation. Stomata are small pores bounded by a pair of guard cells on plant leaf surfaces that regulate carbon uptake and water loss of terrestrial plants [1] . Stomatal conductance ( g s ), determined by stomatal pore aperture and density, has long been a fundamental parameter of earth system models [2] . As g s is sensitive to various environmental change factors, its dynamics are essential for understanding and modeling global carbon and water cycles in a changing climate [3] , [4] . Despite our knowledge about how stomata are regulated by global change factors (GCFs) such as elevated carbon dioxide (CO 2 ) [5] , [6] , [7] , [8] , [9] , warming [10] , change in precipitation [11] , enhanced nitrogen (N) deposition [12] and surface ozone (O 3 ) pollution [13] , [14] (Fig. 1 ), our ability to predict g s in the future is still limited due to three main concerns. First, stomatal sensitivities to different GCFs (e.g., the percentage change of g s per 100 ppm CO 2 increase) remain largely unknown. This is in part due to the fact that the climate forcing used in many manipulation experiments (particularly in the precipitation and nitrogen deposition experiments) exceeded the Intergovernmental Panel on Climate Change (IPCC) predicted ranges [15] , thus suggesting that the stomatal sensitivities normalized to the forcing factor, rather than the overall magnitude of changes, provide more meaningful information for models [16] . Second, the interaction of these g s sensitivities with climate and plant attributes remains poorly understood, limiting our predictive capacity to broad groups of plants having common features (i.e., biomes or plant functional types). Although g s has been related to natural climate gradients [3] , this does not mean that space-for-time substitution can inform how g s will change in the future. Third, there is a paucity of evidence for the g s response to interactions between GCFs, despite their importance for predicting g s in the real world where multiple GCFs are simultaneously in play (e.g., warming × elevated CO 2 concentration) [17] . Empirical data from manipulative experiments will better inform land surface models, such as the Community Atmosphere Biosphere Land Exchange (CABLE) model [18] , if these limitations are resolved. Current land surface models commonly predict g s from net leaf photosynthesis using the Ball-Berry model, which has considered the effects of atmospheric CO 2 concentration but neither the interactions between GCFs nor the differential responses across plant functional types or biomes [2] . Fig. 1: A conceptual diagram depicting the physiological mechanisms underlying the effects of global change factors on stomatal conductance ( g s ). +, –, and ? indicate positive, negative, and uncertain effects, respectively. C i : intercellular CO 2 concentration, ABA: abscisic acid, ROS: reactive oxygen species, VPD: vapor pressure deficit. Full size image Here we synthesized experimental data from 616 published papers to examine the responses of g s to different GCFs, including elevated CO 2 concentration (eCO 2 ), elevated temperature (eT), increased/decreased precipitation (iP/dP), elevated nitrogen deposition (eN), and elevated O 3 concentration (eO 3 ), both individually and in combination. Unlike most previous meta-analyzes [7] , [19] , [20] , [21] , [22] , [23] , [24] , [25] , [26] , we focused on the stomatal sensitivity to various GCFs in addition to the overall magnitude of change. Then, we examined whether the responses of g s to the two-factor combinations were additive, synergistic, or antagonistic. We ultimately predicted the changes in g s by the end of this century across biomes under different scenarios of greenhouse gas emissions [15] , based on the stomatal sensitivities to different GCFs. We found that the GCFs’ effects were commonly additive but became antagonistic as their effect sizes increased. Furthermore, our analysis suggests that rising CO 2 and warming will likely have dominant impacts on the future change in plant gs across biomes. Overview of the global change experiments Our dataset included 5352 pairs of treatment versus control observations for 444 species across different vegetation biomes (Supplementary Data 1 ). The manipulative experiments were mainly conducted in temperate biomes of the Northern Hemisphere in the United States, Europe, and China. The experiments were less common in tropical and subtropical forests (Fig. S 1a ). The treatment magnitudes of eCO 2 and outdoor eT experiments were within the change ranges projected under all the RCPs (Fig. S 1b, c ). In contrast, the magnitudes of iP/dP, eN, and eO 3 were generally greater than the projected ranges from IPCC predictions (Fig. S 1d–g ). Stomatal responses to single global change factors Stomatal conductance was reduced significantly by eCO 2 , eT, dP, and eO 3 , changing on average by –8.3% per 100 ppm CO 2 increase, –1.5% per 1 °C temperature increase, –3.5% per 10% precipitation decrease, and –2.1% per 10 ppb O 3 increase (Fig. 2 ). By contrast, g s was enhanced significantly by iP and eN, with sensitivities of +2.1% per 10% precipitation increase and +0.8% per 1 g m –2 year –1 nitrogen increase (Fig. 2 ). Fig. 2: Responses of g s to global change factors (GCFs). a The overall changes of g s in response to GCFs. b The g s sensitivities in response to GCFs. \(\triangle\) in ( b ) represents one unit of eCO 2 (100 ppm increase), eT (1 °C increase), iP/dP (10% change), eN (1 g m –2 yr –1 increase), or eO 3 (10 ppb increase). The weighted mean values are reported with error bars indicating the 95% confidence interval. All the responses are significantly different from zero at P < 0.05. The numbers outside and inside parentheses represent the number of species ( n sp ) and observations ( n ob ), respectively. See Fig. 1 for variable abbreviations. Full size image The overall magnitudes of changes were significantly greater for the indoor CO 2 , dP, and eN experiments than for the outdoor ones (Fig. S 2a ), but the stomatal sensitivities did not significantly differ between the indoor and outdoor experiments (Fig. S 2b ). The overall change magnitudes increased significantly with the treatment magnitudes for eCO 2 , eT, dP, and eO 3 experiments (Fig. 3a, b, d, f ). The reductions of g s peaked at ΔCO 2 of ca . 300 ppm (Fig. 3a ) or ΔO 3 of 50 ppb (Fig. 3f ), and the stomatal sensitivity decreased significantly with the treatment magnitude of CO 2 , N, and O 3 (Fig. 3g, k, l ). The g s response ratio did vary significantly with experimental duration under eCO 2 (Fig. S 3a ) because the short-term eCO 2 experiments commonly exerted greater treatment magnitudes than the longer-term ones. However, the g s sensitivity did not vary significantly with eCO2 experimental duration (Fig. S 3g ), and the g s responses to other GCFs did not vary with experimental duration (Fig. S 3 b–f, h– 1 ). The response ratios of g s changed significantly with ambient g s under all GCFs except eT (Fig. 4a–f ). The g s sensitivities to eCO 2 and eO 3 were significantly higher for greater ambient g s (Fig. 4g, l ), and the sensitivities to iP and eN were higher for smaller ambient g s (Fig. 4i, k ). The g s responses increased significantly with mean annual temperature under eCO 2 but no other GCFs (Fig. S 4 ). The g s responses to eCO 2 , eT, and dP did not change with aridity index (AI; Fig. S 5a, b, d, g, h, j ), both the response ratio and sensitivity to iP decreased with increasing AI (Fig. S 5c, i ), and the response ratios varied significantly but the sensitivities did not vary with AI under eN and eO 3 (Fig. S 5 e, f, k, 1 ). However, vapor pressure difference (VPD) did not affect the stomatal response ratio or sensitivity to any of the global change factors (Fig. S 6 ). Fig. 3: Stomatal responses to global change factors in relation to treatment magnitude. a – f Natural log-transformed response ratio (ln RR ) of g s to GCFs. g – l Natural log-transformed sensitivity (ln Sens ) of g s to GCFs. The size of each point represents the adjusted weight of each data point, and the darker the color means the higher the point density. The error bands surrounding the regression lines represent the 95% confidence interval. See Fig. 1 for variable abbreviations. Full size image Fig. 4: Stomatal responses to global change factors in relation to plant ambient g s . a – f Natural log-transformed response ratio (ln RR ) of g s to GCFs. g – l Natural log-transformed sensitivity (ln Sens ) of g s to GCFs. The size of each point represents the adjusted weight of each data point, and the darker the color means the higher the point density. The error bands surrounding the regression lines represent the 95% confidence interval. See Fig. 1 for variable abbreviations. 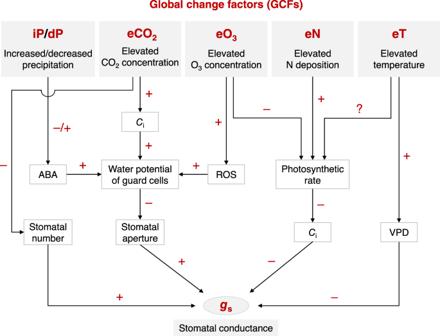Fig. 1: A conceptual diagram depicting the physiological mechanisms underlying the effects of global change factors on stomatal conductance (gs). +, –, and ? indicate positive, negative, and uncertain effects, respectively.Ci: intercellular CO2concentration, ABA: abscisic acid, ROS: reactive oxygen species, VPD: vapor pressure deficit. Full size image The stomatal sensitivities differed significantly among vegetation biomes (Table 1 ) and plant functional types (Table S1 ). Most biomes showed significant sensitivity to eCO 2 , except boreal forest, which only showed significant sensitivity to eT, and Mediterranean woodland, which was not sensitive to any of the tested GCFs (Table 1 ). Only desert plants showed significant sensitivity to iP (Table 1 ). Conifers showed a lower sensitivity to eCO 2 than broad-leaved trees, grasses and forbs (Table S1 ). Table 1 Global environmental change sensitivity of stomatal conductance across biomes Full size table Interactions between global change factors The GCFs’ effects can be additive, antagonistic, or synergistic according to whether the combined effect size is equal, smaller, or larger than the sum of the individual effect size (Fig. S 7 ). All two-factor combinations of GCFs significantly reduced g s except eT+eN, which did not significantly change g s (Fig. 5a ). The interactions between iP and other GCFs were unable to test due to data availability. The individual effects were commonly additive as most points fell around the 1:1 line, but tended to be antagonistic with increasing effect sizes, where the combined effect sizes were smaller than the sum of the individual effect sizes (Fig. 5b ). Fig. 5: Interactive effects between global change factors on g s . a The overall changes of g s in response to two-factor combinations. The error bars represent ±95% of the confidence interval for the weighted means with filled and open points indicating significant ( P < 0.05) and insignificant ( P > 0.05) differences from zero, respectively. The numbers outside and inside parentheses represent the number of species ( n sp ) and observations ( n ob ), respectively. b Relations between ln RR (natural log-transformed response ratio) of two-factor combination and sum of ln RR of the corresponding individual factor. The error bands surrounding the regression lines represent the 95% confidence interval. See Fig. 1 for variable abbreviations. Full size image Future changes in stomatal conductance We examined how individual GCFs alone might change the g s of terrestrial plants by the end of this century based on the predicted magnitudes of changes in different GCFs and the stomatal sensitivities revealed in this study. Under the sustainable emission scenario (SSP1-2.6/RCP2.6), eCO 2 would significantly reduce g s for temperate forests, subtropical forests, temperate grassland, and desert plants, with reduction magnitudes ranging from 4.3% to 9.5% (Fig. 6a ). eT would significantly reduce g s for boreal forest and temperate grassland by 84.8% and 33.1%, respectively (Fig. 6b ). Compared with eCO 2 and eT, the effects of changed precipitation, eN, and eO 3 on g s would be rather small (Fig. 6c–e ). The relative impacts of GCFs were consistent across scenarios (Figs. S 8 and 9 ), i.e., rising CO 2 and warming would dominate future changes in g s across biomes. Fig. 6: Predicted changes in g s across biomes by the end of the twenty-first century under the sustainable emission scenario (SSP1-2.6/RCP2.6). a Changes induced by elevated CO 2 . b Changes induced by warming. c Changes induced by changed precipitation. d Changes induced by elevated N deposition. e Changes induced by elevated O 3 . The left panels display global maps depicting changes in g s , with grey and white land colors indicating areas where changes are statistically insignificant and where is a lack of data, respectively. The right panels depict biome-level predictions, with error bars representing the 95% confidence interval. The numbers outside and inside parentheses represent the number of species ( n sp ) and observations ( n ob ), respectively. Bor.F: boreal forest, Tem.F: temperate forest, Sub.F: subtropical forest, Trop.F: tropical forest, Tem.G: temperate grassland, Med.W: Mediterranean woodland. 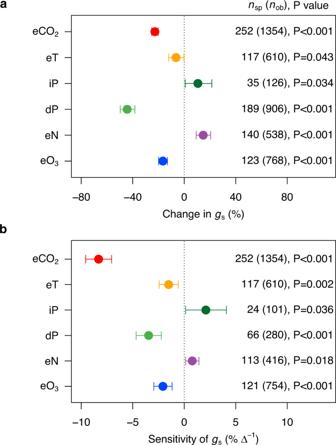Fig. 2: Responses ofgsto global change factors (GCFs). aThe overall changes ofgsin response to GCFs.bThegssensitivities in response to GCFs.\(\triangle\)in (b) represents one unit of eCO2(100 ppm increase), eT (1 °C increase), iP/dP (10% change), eN (1 g m–2yr–1increase), or eO3(10 ppb increase). The weighted mean values are reported with error bars indicating the 95% confidence interval. All the responses are significantly different from zero atP< 0.05. The numbers outside and inside parentheses represent the number of species (nsp) and observations (nob), respectively. See Fig.1for variable abbreviations. Full size image The land surface component of fully coupled climate-carbon cycle models is highly sensitive to the stomatal formulation [27] , [28] . Hence understanding the stomatal response of terrestrial plants to global change is key to improve future coupled water and carbon cycle predictions. Recent meta-analyzes have provided important perspectives on the stomatal response to several GCFs, including eCO 2 [7] , [19] , [20] , [21] , [22] , [24] , eN [23] , and eO 3 [25] , [26] . Our global data synthesis quantified the stomatal responses to five major GCFs across vegetation biomes and revealed two main findings to improve our understanding of stomatal response to global change. First, we showed that the effects between GCFs were commonly additive but tended to be antagonistic as effect sizes increased. Second, we demonstrated that rising CO 2 and warming would dominate future changes in g s across biomes. The overall response patterns of g s to various GCFs are generally consistent with theory predictions shown in Fig. 1 . A recent study showed that g s responses to eCO 2 can be predicted by the optimal stomatal theory, which holds that plants regulate stomata to maximize photosynthesis and minimize water transpiration to achieve optimal water use efficiency [29] . In the past decades, the decline of g s is one of the most consistent responses of plants to eCO 2 that has been documented [7] , [8] , [20] , [21] , [22] . The eCO 2 can reduce g s by decreasing stomatal aperture in the short term and/or stomatal density and size in the long term [5] , [7] , but long-term eCO 2 does not necessarily reduce stomatal density [30] . It has been illustrated that, even though the relative contributions of changes in stomatal aperture vs changes in stomatal density and size differed, short-term and long-term eCO 2 resulted in similar g s responses [6] , in line with our result that g s sensitivity did not vary with experimental duration (Fig. S 3g ). We found that conifer trees exhibited the lowest sensitivity to eCO 2 compared to other plant functional types, in line with previous findings that the stomata of gymnosperm trees were less sensitive to eCO 2 [31] . This pattern was associated with their overall lower ambient g s , because stomatal sensitivity to eCO 2 declined significantly with decreasing ambient g s (Fig. 4g ). As stomata respond to CO 2 concentration at the intercellular space rather than the leaf surface [32] , it is reasonable that plants with higher ambient g s responded more strongly to eCO 2 because it allows more gases to enter and lead to greater increases of CO 2 in the intercellular space. The lower stomatal sensitivity of conifers to eCO 2 and the pattern that stomatal sensitivity reduced with decreasing mean annual temperature (MAT, Fig. S 4g ) together explained why g s of boreal forests were not sensitive to eCO 2 (Table 1 ). Warming is considered to affect plant g s indirectly via Rubisco activity ( V cmax , and consequently photosynthesis and its linkage to g s ), vapor pressure deficit (VPD), and plant water status [10] . Both consistent [33] and inconsistent [34] changes between g s and V cmax have been reported, and warming could change g s independently with VPD in some species [35] , suggesting complex interactions among these mechanisms. It has been proposed that with increasing temperature, g s first increases and peaks at an optimal temperature and then decreases at high temperature [10] . Since the differences between optimal temperatures and growth temperatures might vary with biomes [36] , the response of plant g s to warming is difficult to predict from theory. Here our meta-analysis revealed that warming overall significantly reduced g s (Fig. 2 ), and boreal forests showed the highest sensitivity to eT (Table 1 ). As mentioned above, it should be noted that lowered g s under eT were linked to lowered photosynthetic rates in some but not all cases [37] , [38] . Stomatal responses to changed precipitation are mainly regulated by abscisic acid [11] . In line with the theory prediction, iP (increased precipitation) significantly enhanced g s and dP (decreased precipitation) decreased it. However, there were no significant differences in the stomatal sensitivity to dP among biomes, while the stomatal sensitivity to iP varied significantly across biomes (Table 1 ). Plants grown in drier habitats with lower ambient g s were more sensitive to iP (Figs. 4i and S 5i ) but showed no differences in the sensitivity to dP (Figs. 4j and S 5j ). The results suggest that stomatal sensitivities across biomes are convergent in the responses to drought while divergent in the responses to increased precipitation. The effect of eN on plant g s is most likely indirect, and recent studies suggest two potential mechanisms. First, higher N availability stimulates plant g s as a byproduct of enhanced photosynthetic rate, as evidenced by a positive correlation between the responses of these two traits under eN [23] . Second, N enrichment might deplete soil cations including calcium, which is important for the control of the stomatal aperture [39] . Our results showed that eN significantly increased plant g s , with a threefold greater enhancement for the indoor than the outdoor experiments (Fig. S 2a ). A previous meta-analysis showed that compared with field experiments, indoor N addition induced a twofold greater enhancement of plant biomass [40] , suggesting that indoor N addition stimulated photosynthetic rate and, as a byproduct, plant g s to a greater magnitude. Elevated O 3 may reduce g s directly via producing reactive oxygen species that actively participate in the regulation of the stomatal aperture [13] , [25] or indirectly as a symptom of a decline in photosynthetic rate [14] . Our findings that eO 3 significantly reduced g s confirm previous results of meta-analyzes [25] , [26] . Besides, the result that plants with greater ambient g s were more sensitive to eO 3 (Fig. 4l ) can be explained by a unifying theory, which proposes that cumulative uptake of O 3 into the leaf universally controls the responses of plants (including photosynthesis and growth) across plant functional types [41] . Accordingly, greater treatment magnitude and ambient g s , both facilitating the cumulative uptake of O 3 , are more likely to result in larger stomatal responses. In the real world, different GCF combinations might occur in a given terrestrial ecosystem, but any GCFs will co-occur with eCO 2 [42] . 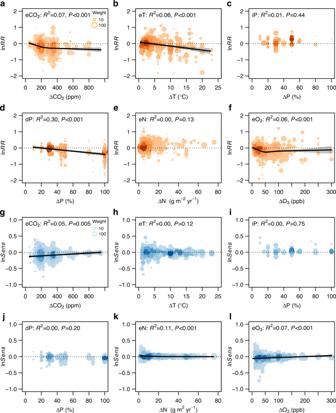Fig. 3: Stomatal responses to global change factors in relation to treatment magnitude. a–fNatural log-transformed response ratio (lnRR) ofgsto GCFs.g–lNatural log-transformed sensitivity (lnSens) ofgsto GCFs. The size of each point represents the adjusted weight of each data point, and the darker the color means the higher the point density. The error bands surrounding the regression lines represent the 95% confidence interval. See Fig.1for variable abbreviations. For combined eCO 2 and other GCFs, their effects on g s were commonly additive but tended to be antagonistic when the effect sizes became larger (Fig. 5b ). The result indicates that eCO 2 might partly diminish the effect of other GCFs on stomata. For instance, it is possible that the lowered g s caused by eCO 2 reduced the uptake and thus the negative impact of O 3 [41] . Similar to our results, prior studies also showed that the GCFs’ effects tended to be antagonistic as the effect sizes became larger for plant biomass [43] , plant N:P ratio [44] , and plant diversity [45] . Interestingly, all these studies used the same method (i.e., paired meta-analyzes), and different methods might lead to contrasting conclusions. For example, studies using Hedges’ d method reported that GCFs’ effects on plant biomass and carbon storage were overall additive [15] , [46] . The Hedges’ d method did not reveal how the interactions vary with effect sizes [44] . The results highlight the importance of the analytical method and imply that models might overestimate the global change effects if additive effects among GCFs are assumed when the effect sizes become larger. Among the GCF combinations we evaluated, how eCO 2 interacts with eN and dP is of particular interest. First, the progressive nitrogen limitation hypothesis proposes that available nitrogen becomes increasingly limiting under eCO 2 as it is sequestered in long-lived plant biomass and soil organic matter [47] . Our dataset cannot directly test this hypothesis, but we found interesting interactions between eCO 2 and eN. Although eN alone significantly increased g s , combined eN and eCO 2 significantly decreased it (Figs. 2 a and 5a ), suggesting that eCO 2 overrode the effect of eN on g s . The results highlight the importance of expanding global change experiments from single to multiple factors in interaction, especially when the effects conflict between GCFs as they did between eCO 2 and eN. Second, there is a long-standing hypothesis that rising CO 2 will ameliorate the impact of drought on plants [48] . Water saved by having lower g s under eCO 2 in the initial period of drought can be used to keep stomata open longer, for photosynthesis in the later phase of drought [49] . Therefore, g s under eCO2+dP may decline less rapidly and transform from being lower to being higher than under dP alone with time. Some studies did show greater g s under eCO 2 + dP than under dP alone [50] , [51] . However, the water-saving effect of eCO 2 at the ecosystem scale, if any, would be smaller than the g s response at the leaf scale, which is often related to the stimulation of the leaf area index (LAI) of the canopy [17] . Besides, we argue that although eCO 2 may save water during the initial phase of drought [52] , it might inversely increase water loss as drought persists. One reason for this is that under severe droughts, plants continue to lose water via the leaf cuticle and incompletely closed stomata in spite of predominately closed stomata. Hence, water loss from leaves continues through minimum leaf conductance ( g min ) rather than mean g s [53] . As LAI would increase under eCO 2 [54] , canopy water loss might also increase if g min is not affected. Secondly, though not directly addressed in most experiments, species competition for survival during water-limited periods might involve water use rather than water savings [55] , [56] . Together, the findings involving eCO 2 interactions with eN and dP support an imperative for future experiments to further address interactions with eCO 2 in large-scale manipulations. Compared with other GCFs, rising CO 2 and warming would exert a greater effect on g s across biomes in the future (Fig. 6 ). This is due to the greater g s sensitivity to eCO 2 and eT (Table 1 ), as well as greater predicted change magnitude in CO 2 concentration by the end of this century [42] , [57] . Under SSP2-4.5 and SSP5-8.5, a few values of predicted g s change magnitude in Figs. S 8 and 9 are unreliable for several biomes, including boreal forests, which may be related to the nonlinear response patterns to eCO 2 [6] , [19] , [58] and eT [10] . Overall, we found that g s was reduced nonlinearly with increasing CO 2 (Fig. 3a ) and the g s sensitivity decreased gradually with rising CO 2 (Fig. 3g ), suggesting a decreasing marginal effect of eCO 2 . The decreasing marginal effect is even more evident when comparing our results from experiments with those from historical records. For example, over the past 150 years, when CO 2 was increased from 290 ppm to 390 ppm, g s was reduced by 34% per 100 ppm CO 2 increase for plants grown in Florida [59] , while in the eCO 2 experiments where CO 2 was on average increased from 370 ppm to 700 ppm, g s was reduced by only 8.2% per 100 ppm CO 2 increase. However, for the warming experiments, we could not derive a nonlinear relationship between g s and temperature [60] . For the boreal forest biome, the g s sensitivity to eT was derived from relatively low warming magnitudes (0.7–1.3 °C); such sensitivity may not be applied to future warming magnitudes under SSP2-4.5 (2.0–7.3 °C) and SSP5-8.5 (3.7–12.5 °C). Besides, due to the same reason, the prediction that eT would reduce the g s of boreal forests by 84.8% under SSP1-2.6 with warming magnitudes of 1.1–5.3 °C (Fig. 6b ) should be employed with caution. The results highlight the importance of dose-response curves between g s and GCFs for predictions, which represent significant challenges for future global change manipulations since the cost of covering a wider treatment range of GCFs will be much higher. Stomatal conductance plays a critical role in plant carbon and water flux. Earth system models integrating the stomatal responses to CO 2 yielded very different projections of future global patterns of precipitation [61] and river runoff [62] . Our findings can inform models by providing stomatal sensitivities of different biomes and plant functional types to major GCFs. Another implication of our results for models is that co-occurring eCO 2 and other GCFs would exert antagonistic effects on g s when the effect sizes become larger, and the combined effects would be overestimated if additive effects are assumed. There are mainly three limitations to the current data synthesis. First, global change experiments are rare in tropical forests, although they represent the most important biomes impacting global carbon and water cycles and have been shown to be sensitive to global changes [15] . While the Coupled Model Intercomparison Project Phase 5 (CMIP5) models assume a great stomatal sensitivity to eCO 2 in tropical regions [63] , empirical data remain lacking. Second, experiments with three or more GCFs are needed to confirm and expand the generality of the g s response patterns observed here. But our results also highlight the influences of rising CO 2 and temperature, suggesting that future studies would need to focus on the overall or net effects of climate change drivers on g s . Third, dose-response curves are critical for accurately predicting future g s under different emission scenarios, but we could only derive an average dose-response curve between g s and eCO 2 based on current data. Thus a great challenge for future global change manipulations would be investigating the dose-response curves for different GCFs across species and biomes. Resolving these limitations in future experiments will significantly improve our understanding and prediction of g s and terrestrial carbon and water cycling in a changing climate. Data sources and compilation Published papers that reported g s responses to GCFs were searched in Web of Science, using the following keywords: TS = (stomatal conductance OR gs) AND TS = (carbon dioxide OR CO2 OR warming OR increasing temperature OR elevated temperature OR precipitation OR rainfall OR drought OR water stress OR nitrogen deposition OR N deposition OR nitrogen addition OR N addition OR ozone OR O3). In addition, papers cited in previous reviews and meta-analysis articles that studied plant responses to global changes were also surveyed. All the papers were further selected by two steps (Fig. S 10 ), and finally, 616 articles (Supplementary References) that met the following criteria were included in the data synthesis: Studies were conducted in terrestrial ecosystems, including forests, deserts, grasslands, and croplands. Both outdoor and indoor studies were included as the g s sensitivities were not significantly different between the two experimental approaches (Fig. S 2 ). However, only the outdoor studies were included when analyzing the g s responses across biomes and the relationships with climates because, for the indoor studies, plants were grown in a controlled environment and thus did not reflect the influence of the local climates. Studies examined the effects of simulated GCFs (i.e., eCO 2 , eT, iP/dP, eN, eO 3 ), individually or in combination. Each study must include control and treatment groups representing the current and future environment, respectively. For instance, experiments had different N input levels but using artificially potting soil (i.e., the mixture of sand, clay, and vermiculite, etc.) or adding P/K (or Hoagland’s solution) were excluded because they could not represent the effects of N deposition on natural ecosystems. g s was measured as mole H 2 O of flux per unit of leaf area (mol m −2 s −1 ) under certain reference conditions (i.e., near-saturation light intensity, treatment-depended CO 2 concentration and temperature, and prevailing humidity) using infrared gas analyzers such as LI-6400/6800 (LI-COR, Lincoln, USA), CIRAS-2/3 (PP Systems, Hitchin, UK), and LCA-2/3/4 (ADC-Biosciences, Hoddesdon, UK). Studies reported the mean values and standard errors of g s of both control and treatment groups with at least three replicates ( n ≥ 3). Data were extracted from the tables, figures, text, and supporting information of the source papers. The Web Plot Digitizer ( https://apps.automeris.io/wpd ) was used to extract data from figures. All relevant observations provided by the source papers were extracted. Observations from different sites or species were considered independent, but multiple observations of the same species at the same site were considered non-independent and treated using the “shifting the unit of analysis” approach (see Text below). Experimental factors which might affect the g s responses including treatment magnitude and experimental duration were also extracted. Basic climatic parameter values (MAT, AI, and water vapor pressure (VP)) were obtained from Worldclim ( http://www.worldclim.org ) based on the site locations if site climate information was not provided in the source papers. VP at saturation (VPsat) was calculated as \(a\times {{{{{\rm{exp }}}}}}\left[b\times {{{{{\rm{T}}}}}}/\left(c+{{{{{\rm{T}}}}}}\right)\right]\) , where a , b , c , and T are constants of 0.611 kPa, 17.502 (unitless), 240.97 °C, and monthly air temperature, respectively, and \({{{{{\rm{VPD}}}}}}={{{{{\rm{VPsat}}}}}}-{{{{{\rm{VP}}}}}}\) . According to the classification of the Koppen-Geiger climatic zones, the biomes of outdoor experiments were categorized into boreal forest, temperate forest, subtropical forest, tropical forest, temperate grassland, Mediterranean woodland, desert, or cropland based on the site locations using the R package ‘kgc’ ( https://cran.r-project.org/web/packages/kgc/ ). Plant species were classified into eight plant functional types: conifer, deciduous broad-leaved tree, evergreen broad-leaved tree, shrub, C3 grass, C4 grass, legume forb, or nonlegume forb. All data used in this study can be accessed in the Supplementary Data file. Meta-analysis The effect size was estimated using the natural log-transformed response ratio ( \({{{{\mathrm{ln}}}}}{RR}\) ) [64] : 
    lnRR=ln(X_T/X_C)
 (1) with a variance of: 
    v_lnRR=SE_T^2/X̅_T^2+SE_C^2/X̅_C^2+τ^2
 (2) where \({\bar{X}}_{{{\mbox{T}}}}\) (and \({{SE}}_{{{\mbox{T}}}}\) ) and \({\bar{X}}_{{{\mbox{C}}}}\) (and \({{SE}}_{{{\mbox{C}}}}\) ) represent the mean (and standard error) of the treatment and control group, respectively; \({\tau }^{2}\) was the between-studies variance and estimated using the R package ‘metafor’ 3.0-2 [65] . The original weighting factor ( w ) of each effect size was given as [64] , [65] : 
    =1/_ln
 (3) When calculating the overall response ratio, the unit of analysis was a species in a site, that is, multiple observations for the same species in the same site were considered non-independent. A “shifting the unit of analysis” method [66] was used to take this non-independence into account. Specifically, the non-independent response ratios were averaged within species within sites, by adjusting the weight of each effect size as [23] , [67] : 
    w^∗=w/n_ob
 (4) where \({w}^{*}\) was the adjusted weighting factor of each effect size, n ob was the total number of observations for the same species at the same site. The overall g s response was quantified using the weighted mean response ratio ( \(\overline{{{{{{\rm{ln}}}}}}RR}\) ): 
    lnRR=∑_i=1^mw_i ^∗×lnRR_i/∑_i=1^mw_i^∗
 (5) where m was the total number of observations for a given GCF or GCFs combination, \({{{{{{\rm{ln}}}}}}{{{{{\rm{RR}}}}}}}_{i}\) and \({w}_{i}^{*}\) were the natural log-transformed response ratio and the adjusted weighting factor of the i th observation, respectively. The standard error of \(\overline{{{{{{\rm{ln}}}}}}RR}\) was calculated as: 
    SE_lnRR=√(1/∑_i=1^mw_i^∗)
 (6) And the 95% confidence interval (CI) for \(\overline{{{{{{\rm{ln}}}}}}RR}\) was calculated as: 
    95% CI=lnRR± 1.96×SE_lnRR
 (7) The \(\overline{{{{{{\rm{ln}}}}}}RR}\) with 95% CI was estimated with the random-effects model in R using the package ‘metafor’ 3.0–2 [65] . Finally, \(\overline{{{{{{\rm{ln}}}}}}RR}\) was transformed to percentage change (%) as: 
    Percentage  change=(exp (lnRR)-1)× 100
 (8) The impacts of treatment magnitude, plant attributes (ambient g s , vegetation biomes, and plant functional types), and climate on the g s responses were assessed via the meta-regression function of the package ‘metafor’. Both linear and nonlinear regressions were performed, and the nonlinear meta-regressions were conducted by fitting the “restricted cubic splines” model with the additional help of the ‘rms’ package. Results of the better-performed linear or nonlinear regressions with higher R 2 values were reported. The publication bias was evaluated by funnel plots. Funnel plot asymmetry was further tested with Egger’s regression in R using the ‘metafor’ package. Results showed all the studies except eT+dP were distributed symmetrically around the mean effect size in the funnel plots (Fig. S 11 ), suggesting publication bias only might exist in the warming and drought combined experimental data. Stomatal sensitivity to global change factors The natural log-transformed g s sensitivity ( \({{{{\mathrm{ln}}}}}{Sens}\) ) was calculated as [68] : 
    ln Sens=ln RR/
 (9) with a variance of: 
    v_sens=v_RR/^2
 (10) where \({{{{\mathrm{ln}}}}}{RR}\) was the natural log-transformed response ratio, \({v}_{{{\mbox{RR}}}}\) was the variance of \({{{{\mathrm{ln}}}}}{RR}\) , and \(\triangle\) was the treatment magnitude in standardized units [69] . Here, the absolute magnitudes were used for eCO 2 (per 100 ppm increase), eT (per 1 °C increase), eN (per 1 g m –2 yr –1 increase), and eO 3 (per 10 ppb increase), and the relative magnitude was used for iP/dP (per 10% change), according to previous studies [15] , [68] . The weighted means of \({{{{\mathrm{ln}}}}}{Sens}\) and percentage sensitivity were calculated similarly to the \(\overline{{{{{{\rm{ln}}}}}}RR}\) (Eq. 5 ) and \({{{{{\rm{Percentage}}}}}}\;{{{{{\rm{change}}}}}}\) (Eq. 8 ) above. Interactions between global change factors The interactions were evaluated via paired meta-analyzes, a conservative approach by comparing the effect size of combined factors with the sum of effect sizes of the corresponding individual factors [43] , [44] . For positive summed effect sizes, the synergistic, antagonistic, and additive interactions should fall above, below and on the 1:1 line, corresponding to larger (more positive), smaller (less positive), and equal combined effect sizes. For negative summed effect sizes, the synergistic, antagonistic, and additive interaction should fall below, above, and on the 1:1 line, corresponding to larger (more negative), smaller (less negative), and equal combined effect sizes, respectively (Fig. S 7 ). Impacts of future global change The global change impacts on g s by the end of the twenty-first century were evaluated by multiplying the g s sensitivities with the projected change magnitudes of GCFs under different emission scenarios. To make the predictions spatially explicit, we used the biome-specific g s sensitivities (Table 1 ) combined with maps of global changes in different GCFs. For atmospheric CO 2 concentrations, present and future conditions were produced by averaging data from the Mauna Loa Observatory, Hawaii ( http://CO2now.org ) for the period 1981–2000 and the SSP Database ( https://tntcat.iiasa.ac.at/SspDb/ ) for the period 2081–2100, respectively (Table S2 ). For temperatures and precipitations, the bioclimatic variables ‘mean annual temperature’ (BIO1) and ‘annual precipitation’ (BIO12) in the WorldClim v2.1 climate database ( https://worldclim.org ) were used. In WorldClim, present and future conditions were produced by averaging historical data for the period 1970–2000 and averaging data from eight general circulation models (GCMs) (Table S2 ) for the period 2081–2100, respectively. For N depositions, average values from seven models (Table S2 ) of the Coupled Model Intercomparison Project Phase 6 (CMIP6) datasets for the period 1981–2000 and 2081–2100 were used. For ground-level O 3 concentrations, current and future conditions were produced via averaging data from six global atmospheric chemistry transport models (Table S2 ) during a period centered around 2000 and 2100, respectively [70] . Three future Shared Socioeconomic Pathways (SSP) scenarios were used for the predicted future changes in CO 2 concentration, temperature, precipitation, and N deposition: (1) the SSP1-2.6, a sustainable scenario that respects perceived environmental boundaries; (2) the SSP2-4.5, ‘middle of the road’ scenario which emission trends do not shift markedly from historical patterns; and (3) the SSP5-8.5, rapid economic and social development coupled with the exploitation of abundant fossil fuel resources. The SSPs are not yet available for ground-level O 3 , thus the corresponding Representative Concentration Pathway (RCP) scenarios (RCP2.6, RCP4.5, and RCP8.5, respectively) were used. Only the predictions of the direct effects of each GCF on g s were made because there were complex combinations of multiple GCFs in a specific location that were unable to be taken into account using currently available data. The average changes of g s with 95% CI at the biome level were estimated by calculating the average change magnitude of each GCF, and multiplying it by the weighted mean sensitivity with 95% CI of each GCF in Table 1 . 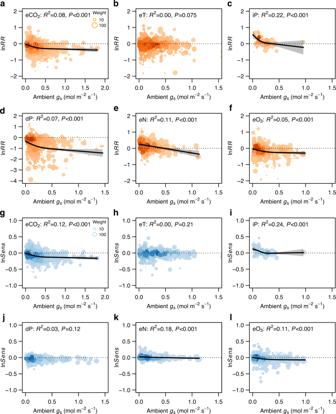Fig. 4: Stomatal responses to global change factors in relation to plant ambientgs. a–fNatural log-transformed response ratio (lnRR) ofgsto GCFs.g–lNatural log-transformed sensitivity (lnSens) ofgsto GCFs. The size of each point represents the adjusted weight of each data point, and the darker the color means the higher the point density. The error bands surrounding the regression lines represent the 95% confidence interval. See Fig.1for variable abbreviations. 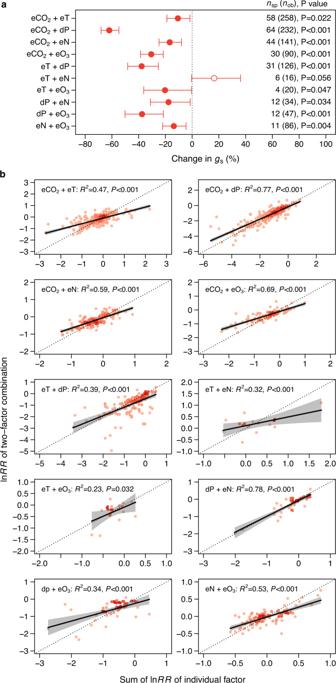Fig. 5: Interactive effects between global change factors ongs. aThe overall changes ofgsin response to two-factor combinations. The error bars represent ±95% of the confidence interval for the weighted means with filled and open points indicating significant (P< 0.05) and insignificant (P> 0.05) differences from zero, respectively. The numbers outside and inside parentheses represent the number of species (nsp) and observations (nob), respectively.bRelations between lnRR(natural log-transformed response ratio) of two-factor combination and sum of lnRRof the corresponding individual factor. The error bands surrounding the regression lines represent the 95% confidence interval. See Fig.1for variable abbreviations. 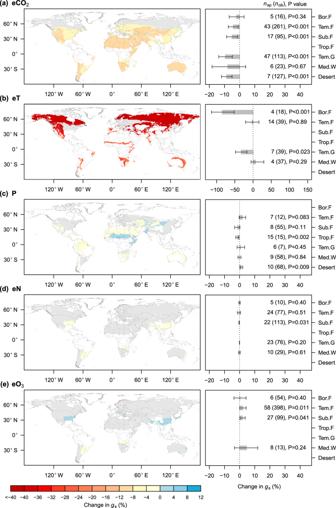Fig. 6: Predicted changes ingsacross biomes by the end of the twenty-first century under the sustainable emission scenario (SSP1-2.6/RCP2.6). aChanges induced by elevated CO2.bChanges induced by warming.cChanges induced by changed precipitation.dChanges induced by elevated N deposition.eChanges induced by elevated O3. The left panels display global maps depicting changes ings, with grey and white land colors indicating areas where changes are statistically insignificant and where is a lack of data, respectively. The right panels depict biome-level predictions, with error bars representing the 95% confidence interval. The numbers outside and inside parentheses represent the number of species (nsp) and observations (nob), respectively. Bor.F: boreal forest, Tem.F: temperate forest, Sub.F: subtropical forest, Trop.F: tropical forest, Tem.G: temperate grassland, Med.W: Mediterranean woodland. Reporting summary Further information on research design is available in the Nature Portfolio Reporting Summary linked to this article.